Bio-inspired nanocatalysts for the oxygen reduction reaction Electrochemical conversions at fuel cell electrodes are complex processes. In particular, the oxygen reduction reaction has substantial overpotential limiting the electrical power output efficiency. Effective and inexpensive catalytic interfaces are therefore essential for increased performance. Taking inspiration from enzymes, earth-abundant metal centres embedded in organic environments present remarkable catalytic active sites. Here we show that these enzyme-inspired centres can be effectively mimicked in two-dimensional metal-organic coordination networks self-assembled on electrode surfaces. Networks consisting of trimesic acid and bis-pyridyl-bispyrimidine coordinating to single iron and manganese atoms on Au(111) effectively catalyse the oxygen reduction and reveal distinctive catalytic activity in alkaline media. These results demonstrate the potential of surface-engineered metal-organic networks for electrocatalytic conversions. Specifically designed coordination complexes at surfaces inspired by enzyme cofactors represent a new class of nanocatalysts with promising applications in electrocatalysis. Energy and climate change have become one of the biggest preoccupations attracting the common interest of science, engineering and society. In this important field, electrochemistry provides a bridge for efficient interconversion of chemical to electrical energy, that is, fuel cells [1] , [2] , [3] . Fuel cells based on oxidation of H 2 and reduction of O 2 require electrocatalytic surfaces since the electrode processes are not simple reactions and show a strong dependence on the nature of the electrode material. For instance, a direct relationship between the kinetic rates of the oxygen reduction reaction (ORR) and the surface electrode structure was found for gold single crystals [4] , [5] . ORR is a complex reaction and an effective and inexpensive catalyst that can compete with or exceed the efficiency of platinum remains an ongoing challenge. The physical and economic requirements of low overpotential, long-term stability, pH working conditions, non-toxic and earth-abundant elements, and so on impose severe boundaries on the usable material combinations. Nature provides an alternative and efficient solution to this problem, that is, the O 2 in our atmosphere is biogenic—the result of a catalytic process in the photosynthetic machinery of green plants [6] . With increasing atmospheric oxygen levels, higher life-forms with oxygen-metabolizing enzymes evolved. These naturally occurring oxygen activation catalysts, which have been utilized in biological processes for several hundred millions of years, are considered as viable substitutes for precious metals in ORR catalysts for fuel cells [7] , [8] , [9] . Considering both biological and classical inorganic catalysts, one finds close relation between structure and function. In the case of the enzymatic ORR catalysts, nature uses, first, molecules containing electron-donating functional groups that prevent the formation and release of detrimental partially reduced oxygen by-products and intermediates [10] . Second, bulky protein chains sufficiently separate the ORR inorganic active sites, preventing site overlap and catalytic deactivation [9] . The active sites, mostly composed of first-row transition metal atoms and clusters, share a common and important feature with classical inorganic catalysts, that is, the presence of coordinatively unsaturated sites, which play a prominent role in heterogeneous catalytic transformations [11] , [12] . Thus, new catalytic materials can be designed that are inspired by both natural and classical ORR catalysts by using organic molecules with specific molecular backbones (adequately separating the active sites) and selected functional groups (electron withdrawing or donating) to coordinate transition metal atoms or clusters directly on surfaces. Thus, two-dimensional metal-organic coordination networks (2D-MOCNs), that is, organic molecules and metal centres self-assembled on surfaces under well-controlled conditions, constitute a promising route to fabricate functional low-dimensional bio-inspired architectures [13] . 2D-MOCNs were created using organic ligands with different functional groups (carboxylic acid, pyridyl, cyano and hydroxyl end groups) and metal centres (Mn, Fe, Co, Ni and Cu) on various noble metal substrates like Au, Ag, Cu or highly ordered pyrolytic graphite [13] , [14] , [15] , [16] . An example of a 2D-MOCN is presented in Fig. 1 showing a Scanning tunnelling microscopy (STM) image of biphenyl-dicarboxylic acid self-assembled with Fe atoms on Cu(100) [17] . The biphenyl-dicarboxylic acid ligand coordinates with its two-terminal carboxylate groups to dimeric Fe centres, thus forming an extended and periodic 2D coordination polymer. The network presents open cavities where the underlying substrate is exposed. Each network node consists of two coordinatively unsaturated Fe centres with each atom being threefold coordinated to carboxylate oxygen atoms (see Fig. 1 ). The network is chemisorbed to the copper surface but the top binding position of the Fe centres remains open. Moreover, the hybridization of the metal centres with the metal surface is significantly reduced yielding atomic-like electronic configurations for the Fe ions as found for isolated metal–organic complexes [18] . 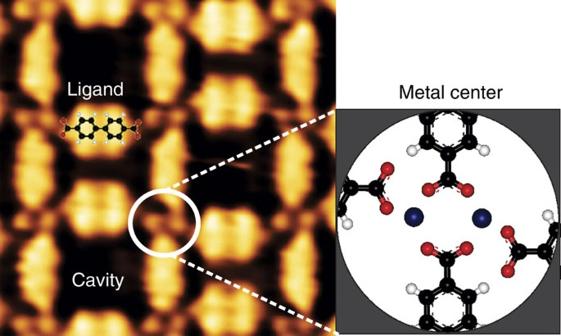Figure 1: Example of 2D-MOCNs. Scanning tunneling microscopy image of Fe-biphenyl-dicarboxylic acid on Cu (100) self-assembled under UHV conditions. The main features of 2D-MOCNs are indicated: metal centre, organic ligand and cavity. The expansion illustrates the Fe coordination environment17. Figure 1: Example of 2D-MOCNs. Scanning tunneling microscopy image of Fe-biphenyl-dicarboxylic acid on Cu (100) self-assembled under UHV conditions. The main features of 2D-MOCNs are indicated: metal centre, organic ligand and cavity. The expansion illustrates the Fe coordination environment [17] . Full size image Engineering of the synthetic ligands in combination with the judicious choice of the metal centres and substrates allows complete control on the network structure, separation and coordination geometry of the metal centres as well as the size of the generated cavities [17] , [19] . To date, the most explored application of surface-supported 2D networks so far is the accommodation of guest molecules inside the cavities [20] , [21] . Initial experiments on the reactivity of the metal centres towards O 2 adsorbed from the gas phase [22] indicate the high potential of 2D-MOCNs as tailor-made heterogeneous electrocatalysts. In the present work, we show that rationally designed 2D−MOCN exhibit substantial electrocatalytic activity for the ORR in alkaline media. The electrochemical behaviour differs from bare Au(111) and the ORR mechanism depends strongly on the choice of the metal centre, while the stability of the network is determined by the organic molecule. The networks containing Fe atoms exhibit a (2+2)e − pathway for the complete reduction to H 2 O, while the coordinated Mn atoms show evidence for a direct 4e − route to convert O 2 to H 2 O. Formation of metal–organic networks on Au(111) The networks consist of benzene-1,3,5-tricarboxylic acid (TMA, Fig. 2a ) and Fe or Mn atoms and 5,5′-bis(4-pyridyl)(2,2′-bipirimidine) (PBP, Fig. 2b ) and Fe atoms self-assembled on Au(111). Both carboxylic and pyridyl ligands coordinating Fe and Mn atoms were selected to mimic both biological and inorganic catalysts for ORR [22] , [23] , [24] , [25] . The aromatic rings ensure the planarity of the coordination structure on the surface and define the separation of the reactive metal centres. STM was employed to determine the structural details of the architectures and to confirm the network formation as well as estimate coverage before the electrochemical measurements. Sample preparation and STM characterization are conducted under ultra-high vacuum (UHV) conditions. A sample transfer system connecting the UHV chamber and the electrochemical cell permits full atmospheric control of the sample environment throughout the experiments ( Supplementary Fig. S1 ). 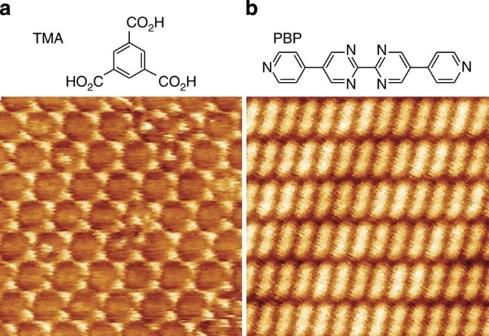Figure 2: Chemical structure and STM topography of the organic ligands on Au(111). (a) STM image (12 × 12 nm2) of the TMA honeycomb network and (b) 8 × 8 nm2STM image of PBP on Au(111). Figure 2: Chemical structure and STM topography of the organic ligands on Au(111). ( a ) STM image (12 × 12 nm 2 ) of the TMA honeycomb network and ( b ) 8 × 8 nm 2 STM image of PBP on Au(111). Full size image 2D networks of TMA were previously investigated on different single crystals by STM in both UHV and liquid environment [26] , [27] , [28] , [29] , [30] . On Au(111), TMA is physisorbed with the aromatic ring orientated parallel to the surface. The carboxyl groups form intermolecular hydrogen bonds resulting in a porous network well-known as ‘honeycomb’ structure, see Fig. 2a . The honeycomb pattern is composed of six bright triangular features representing individual TMA molecules [26] , [27] , [28] , [29] , [30] . After TMA deposition, either Fe or Mn atoms are incorporated into the network (see Methods). During this process, the carboxyl moieties of TMA are expected to deprotonate favouring the O−metal interaction [31] . An STM image of TMA−Fe on Au(111) is shown in Fig. 3a . The TMA−Mn structure is nearly indistinguishable from TMA−Fe ( Supplementary Fig. S2 ). A high-resolution STM image and proposed model are presented in Fig. 3b . Clearly, the motif of the original TMA network changes after the incorporation of metal atoms. On the basis of corresponding systems studied previously, a model is adapted. The confirmation of the stoichiometry and structure is, however, not straightforward. The triangular features are interpreted as flat-lying TMA molecules. Particular regions between the molecules appear brighter and are assigned to the positions of the metal atoms, thereby creating coordination chains where in each segment metal dimers coordinate to four molecules. TMA−Fe networks on other substrates show different arrangements [31] , [32] , [33] , [34] . Here the metal dimers are bridged by two carboxylate groups with each metal atom coordinating to three oxygen atoms. Adjacent coordination chains are potentially interlinked by carboxyl hydrogen bonds, which require only partial deprotonation of TMA. Further information containing unit cell and network dimensions are presented in Supplementary Fig. S3 and Supplementary Table S1 . 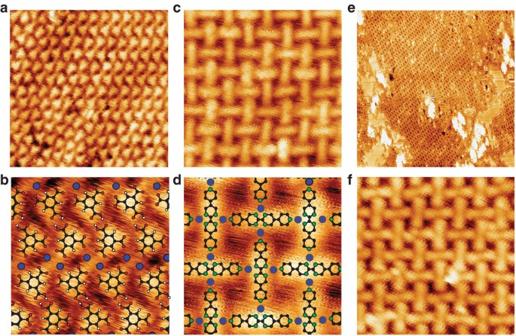Figure 3: STM topography and model of TMA-Fe and PBP-Fe. (a) STM image (12 × 12 nm2) of TMA−Fe network on Au(111). (b) High-resolution (3.75 × 3.75 nm2) STM image of TMA−Fe with the model superposed. (c) STM image (8 × 8 nm2) of PBP−Fe network on Au(111). (d) High-resolution (3.5 × 3.5 nm2) STM image of PBP−Fe with the model superposed. (e) Large-scale (74 × 74 nm2) STM image of PBP−Fe after EC experiments. (f) Zoom ofe: 8 × 8 nm2STM image of PBP−Fe after EC experiments. Colour legend: N (green), C (black), O (red), H (white). H is omitted in PBP scheme. Figure 3: STM topography and model of TMA-Fe and PBP-Fe. ( a ) STM image (12 × 12 nm 2 ) of TMA−Fe network on Au(111). ( b ) High-resolution (3.75 × 3.75 nm 2 ) STM image of TMA−Fe with the model superposed. ( c ) STM image (8 × 8 nm 2 ) of PBP−Fe network on Au(111). ( d ) High-resolution (3.5 × 3.5 nm 2 ) STM image of PBP−Fe with the model superposed. ( e ) Large-scale (74 × 74 nm 2 ) STM image of PBP−Fe after EC experiments. ( f ) Zoom of e : 8 × 8 nm 2 STM image of PBP−Fe after EC experiments. Colour legend: N (green), C (black), O (red), H (white). H is omitted in PBP scheme. Full size image 2D metal-organic networks of PBP have been reported on Ag and Cu surfaces but not on Au(111) [35] . An STM image of the molecular network of PBP on Au(111) is shown in Fig. 2b . On Au(111), PBP adsorb in a flat geometry with the aromatic rings parallel to the surface. A lamellar structure is observed with the molecules oriented parallel and aligned in rows. The pyrimidine groups are adjacent to each other and the pyridyl end groups form hydrogen bonds resulting in a skewed structure. The tilt accounts for a closer proximity and better alignment of the N-functional groups. Similar structures were observed with the pyridyl benzoic acid molecule assembled on Ag(111) [36] and PBP on Ag(100) [35] . On incorporation of Fe, a network structure forms, which is comparable to the networks formed on Cu and Ag surfaces using Cu adatoms [35] . Figure 3c–f shows STM images of PBP−Fe on Au(111) directly after preparation in UHV (c,d) and after the electrochemical (EC) experiments (e and f, see Discussion below). A high-resolution STM image and proposed model are presented in Fig. 3d . In this network, each molecule coordinates to four Fe adatoms via the pyrimidine and pyridyl groups fully saturating the molecule’s binding sites. Hence, each Fe adatom binds to three nitrogen atoms of the two central pyrimidine units of a PBP molecule and to the pyridyl moiety of a neighbouring PBP ligand. Network parameters are presented in Supplementary Fig. S3 and Supplementary Table S1 . Electrocatalytical properties of the networks The presence of precisely defined and coordinatively unsaturated metal atoms (Fe or Mn) opens the possibility to explore the electrocatalytic properties of these nanostructures. Here we explore the ability of the networks to reduce O 2 in alkaline media. 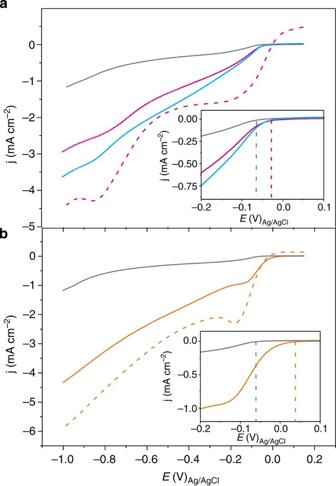Figure 4: ORR polarization curves. Polarization curves in O2-saturated 0.1 M NaOH solution at 0.05 V s−1for: (a) bare Au(111) (grey solid line), TMA−Fe (pink solid line), PBP−Fe (turquoise solid line) and TMA−Fe after the addition of 10 mM H2O2(pink-dashed line); (b) bare Au(111) (grey line), TMA−Mn (orange) and TMA−Mn after the addition of 10 mM H2O2(orange-dashed line). The insets in the graphs show the different onset potential for the shoulder at −0.2 V. On Au(111), the reduction of O 2 occurs via a 2e − pathway with the final product H 2 O 2 ( HO 2 − in basic media) according to the following mechanism [4] , [5] : Figure 4a shows the polarization curve for the bare Au(111) (grey line) in O 2 -saturated 0.1 M NaOH solution. The weak shoulder at −0.20 V with a current density around 0.25 mA cm −2 corresponds to the reduction of O 2 to H 2 O 2 (equation (1)). The polarization curves for TMA−Fe and PBP-Fe acquired under the same conditions are presented in Fig. 4a (pink and turquoise lines). Multiple potential sweeps can be done without major changes proving reversibility ( Supplementary Fig. S4 ). TMA-Fe and PBP-Fe polarization curves differ significantly from bare Au(111). First, the shoulder at −0.2 V shows an onset shifted ~0.05 V to lower overpotentials (see also inset in Fig. 4a ) and has tripled current density (0.75 mA cm −2 ) compared with bare Au(111). Second, and much more striking, is the presence of a second peak at about −0.80 V with a large current density (2.5 and 3 mA cm −2 for TMA-Fe and PBP-Fe, respectively). Small differences are observed between TMA-Fe and PBP-Fe polarization curves. First, PBP-Fe has a somewhat larger catalytic current, which can be related to the higher density of Fe ions ( Supplementary Table S1 ). Second, the position of the peak at about −0.8 V is shifted to more negative potentials for PBP-Fe. This could be a result of the distinct coordination environment. By analogy with other Fe-containing systems, the second shoulder can be assigned to the electroreduction of H 2 O 2 to H 2 O ( OH − in basic media) [37] according to the following reaction: Figure 4: ORR polarization curves. Polarization curves in O 2 -saturated 0.1 M NaOH solution at 0.05 V s −1 for: ( a ) bare Au(111) (grey solid line), TMA−Fe (pink solid line), PBP−Fe (turquoise solid line) and TMA−Fe after the addition of 10 mM H 2 O 2 (pink-dashed line); ( b ) bare Au(111) (grey line), TMA−Mn (orange) and TMA−Mn after the addition of 10 mM H 2 O 2 (orange-dashed line). The insets in the graphs show the different onset potential for the shoulder at −0.2 V. Full size image To test that hypothesis, H 2 O 2 was added to the solution. The polarization curve for TMA-Fe in the presence of 10 mM H 2 O 2 in O 2 -saturated 0.1 M NaOH solution is shown in Fig. 3a (pink-dashed line). Polarization curves for PBP-Fe in the presence of 10 mM H 2 O 2 in O 2 -saturated 0.1 M NaOH give a similar result ( Supplementary Fig. S5 ). The H 2 O 2 electroreduction of TMA-Fe presents two well-defined waves at −0.2 and −0.8 V in the employed potential window, thus confirming the hypothesis. The increase in the current density by adding H 2 O 2 can be traced back to an increase of the surface concentration of O 2 owing to disproportionation of H 2 O 2 in alkaline media [38] . On bare Au(111), a similar pattern is generated ( Supplementary Fig. S6 ) if the potential window is extended to at least up to −1.3 V because the second wave (H 2 O 2 reduction) is shifted to more negative potentials (−1.2 V). This is a significant result as it means that TMA−Fe and PBP-Fe networks also catalyse the decomposition of H 2 O 2 lowering the overpotential by 0.4 V, which is of high importance in biotechnological applications [39] . The ability of Fe to reduce O 2 is widely explored in the literature, and several mechanisms were identified yielding H 2 O or H 2 O 2 as a final product [37] , [40] , [41] , [42] . For TMA−Fe and PBP-Fe networks, we propose that the first wave at −0.2 V in the polarization curve is related to reduction of O 2 towards H 2 O 2 mediated by both exposed Au surface areas and oxygen atoms present in the MOCNs. In fact, the polarization curve for pure TMA or PBP on Au(111) ( Supplementary Fig. S5a,b ) shows a small enhancement of the current density compared with bare Au(111). In UHV conditions, the Fe centres in the network assume an oxidation state close to Fe(II) [18] , [43] , and Fe(II) can readily bind O 2 . However, we do not expect the Fe atoms to participate in the reaction because in the potential window of the first wave between −0.20 and −0.40 V, we assume trivalent metal centres present in the network. It is well established that Fe(III) is not favoured as an active site for O 2 reduction [41] . Analysing the second wave, we consider that Fe(II) species become predominant at potentials more negative than −0.60/−0.70 V. At this potential, Fe(II) can bind both O 2 or H 2 O 2 to form OHOH adducts. The strong bonding of H 2 O 2 to Fe(II) prevents it from leaving as a two-electron reduction product and provides a path for final reduction to H 2 O [41] . The presence of Fe in the TMA and PBP networks explains the second wave, and a mechanism combining equations (1) and (2) is proposed. Blank experiments using the same amount of Fe (0.07 monolayer) contained in the networks deposited on Au(111) at room temperature show a similar behaviour as TMA−Fe and PBP-Fe networks but with substantially reduced catalytic activity ( Supplementary Fig. S5a,b ). The Fe is probably present as small clusters at the elbow sites of the Au(111) herringbone reconstruction. The key role of the unsaturated metal centres in the electrocatalytic reduction of oxygen becomes evident when going from Fe- to Mn-based MOCNs. Figure 4b shows the polarization curve for TMA–Mn (orange-solid line) in O 2 -saturated 0.1 M NaOH solution. A distinct behaviour is observed in comparison with bare Au(111) and TMA-Fe, PBP-Fe networks The first wave is shifted to a lower potential of −0.15 V with an onset potential lowered by 0.1 V (see inset in Fig. 4b ) and presents a high current density (1 mA cm −2 ), which is also better defined. Moreover, the wave at −0.8 V found in both PBP-Fe and TMA−Fe ORR polarization curve is not present for the TMA−Mn network. A possible reason could be that the potential reduction of small amounts of the generated H 2 O 2 is obscured by the onset of the hydrogen evolution reaction. However, adding 10 mM H 2 O 2 to the O 2 -saturated 0.1 M NaOH solution does not produce any change in the shape of the polarization curve (orange-dashed line in Fig. 4b ), indicating that no H 2 O 2 electroreduction occurs. In addition, here we find an increase in the current density by adding H 2 O 2 due to disproportionation of H 2 O 2 in alkaline media as found for the Fe-containing networks [38] . Hence, we conclude that the TMA−Mn network reduces O 2 directly to H 2 O trough a 4e − pathway according to the following equation: It is important to point out that Mn oxides catalyse the O 2 reduction mainly via a (2+2)e − pathway [44] , while Mn coordination compounds [45] directly reduce O 2 to H 2 O via a 4e − mechanism. Similar to Fe on Au(111), the polarization curves for Mn clusters (0.07 monolayers) on Au(111) show a similar profile as TMA−Mn with clearly lower catalytic current density ( Supplementary Fig. S5c ). This result emphasizes the importance of the complexation of the metal atoms and hints at the tremendous potential of this approach. On one hand, the chemical activity of the metal centres is determined by both the nature of the metal ion and its coordination shell. On the other hand, the ligation separates the unsaturated metal atoms preventing catalytic deactivation [9] . Thus, the specific design of ligands allows tuning the catalytic activity of metal adatoms for a desired chemical conversion. Although repetitive EC curves show the reversibility and stability of the system ( Supplementary Fig. S4 ), STM measurements of TMA networks after the EC experiments were difficult to perform probably because of residual adsorbates from the electrolyte solution even after rinsing and drying the sample. Imaging of PBP-Fe networks proved to be less delicate. A large-scale STM image of PBP-Fe after EC measurement is shown in Fig. 3e . The image represents well the system after the EC experiment. First, long-range 2D-network domains are still presented after the EC experiment. Second, a nearly identical structure was found after the liquid environment compared with the UHV-prepared network (see high-resolution image in Fig. 3f ). In addition, some agglomerates are present, which are associated with residual adsorbates from the electrolyte solution. We have demonstrated that 2D-MOCNs of TMA−Fe, PBP−Fe and TMA−Mn on Au(111) catalyse the ORR and, moreover, that the final product and mechanism can be influenced by the choice of the metal centre. While Fe structures exhibit a (2+2)e − mechanism, the TMA−Mn networks can directly reduce O 2 through a 4e − pathway. To obtain deeper understanding of the electron transfer characteristics and to overcome kinetic limitations, a flow-cell system will be implemented in future experiments. This work provides a proof of concept that surface-engineered metal–organic complexes and networks that display structural resemblance with enzyme active sites have a high potential for heterogeneous catalytic chemical conversions. The possibility to create novel and highly stable functional 2D coordination complexes at surfaces using specifically designed organic molecules and transition metal centres taking inspiration from nature opens up a new route for the design of a new class of nanocatalyst materials with promising applications in electrocatalysis. Sample preparation and STM data acquisition Network preparation and STM measurements were conducted in a home-built UHV chamber (base pressure ~5 × 10 −10 mbar). The Au(111) single-crystal substrate (MaTeck) was cleaned by repeated cycles of sputtering with Ar + ions and annealing at 825 K. TMA was purchased from Sigma-Aldrich (purity 97%) and PBP was kindly provided by Professor Mario Ruben [35] . The molecular powders were sublimed from a quartz crucible at 465 and 470 K for TMA and PBP, respectively, onto the surface held at room temperature. For the TMA networks, atomic iron and manganese (purity 99.9%) were evaporated using an electron-beam-heated evaporator. Subsequent to metal evaporation, the substrate was annealed to 525 K resulting in a full monolayer of either TMA−Fe or TMA−Mn. In contrast, pure TMA networks cannot be annealed higher than 353 K because of desorption of the molecules. For PBP networks, atomic iron was evaporated onto the surface held at 413 K resulting in full monolayer network coverage. The STM topographs were acquired at 298 K. WsXM software was used for image analysis [46] . Transfer of the sample from UHV to electrochemical cell A home-built sample transfer system between UHV and EC environment was implemented. Supplementary Fig. S1 shows a scheme of the experimental set-up. After UHV preparation of the sample and verification by STM, the sample was brought to the transfer chamber and a 1-bar Argon atmosphere was established. For the STM characterization of the surfaces after the EC experiments, the sample was removed from the electrochemical cell under potential control (0.15 V), rinsed with water, dried in Ar atmosphere and heated to remove most of the residual adsorbates originating from the electrolyte solution. Electrochemical experiments ORR experiments were carried out in a three-electrode conventional electrochemical cell. The 0.1 M NaOH solution was prepared using NaOH pellets from Sigma-Aldrich (99.99% trace metals basis) and milliQ water (18.2 MΩ). Oxygen and Argon gases were of 5.0 purity. Silver/silver chloride (3 M KCl) and Pt- or Au-coiled wire were used as a reference and counter electrode, respectively. All potentials are referred to the Ag/AgCl/(3 M KCl) reference electrode. Cyclic voltammetry experiments were carried out using an Autolab potentiostat (Ecochemie Inc., model PGSTAT 302N). How to cite this article: Grumelli, D. et al. Bio-inspired nanocatalysts for the oxygen reduction reaction. Nat. Commun. 4:2904 doi: 10.1038/ncomms3904 (2013).